Seeded growth of highly crystalline molybdenum disulphide monolayers at controlled locations Monolayer transition metal dichalcogenides are materials with an atomic structure complementary to graphene but diverse properties, including direct energy bandgaps, which makes them intriguing candidates for optoelectronic devices. Various approaches have been demonstrated for the growth of molybdenum disulphide (MoS 2 ) on insulating substrates, but to date, growth of isolated crystalline flakes has been demonstrated at random locations only. Here we use patterned seeds of molybdenum source material to grow flakes of MoS 2 at predetermined locations with micrometre-scale resolution. MoS 2 flakes are predominantly monolayers with high material quality, as confirmed by atomic force microscopy, transmission electron microscopy and Raman and photoluminescence spectroscopy. As the monolayer flakes are isolated at predetermined locations, transistor fabrication requires only a single lithographic step. Device measurements exhibit carrier mobility and on/off ratio that exceed 10 cm 2 V −1 s −1 and 10 6 , respectively. The technique provides a path for in-depth physical analysis of monolayer MoS 2 and fabrication of MoS 2 -based integrated circuits. The presence of an intrinsic direct energy bandgap in molybdenum disulphide (MoS 2 ) monolayers makes this two-dimensional material of both fundamental and technological interest [1] , [2] , [3] , [4] , [5] , [6] , [7] , [8] , [9] , [10] . Several synthetic methods have been reported, including sulphiding of Mo thin film [11] , and annealing of ammonium tetrathiomolybdate, which has both Mo and S components [12] . One promising technique is the growth of MoS 2 flakes by chemical vapour deposition (CVD) of molybdenum trioxide (MoO 3 ) and solid sulphur, which can yield highly crystalline, predominantly monolayer material [13] , [14] , [15] , [16] , [17] . However, this method typically leads to growth of MoS 2 flakes in uncontrolled locations on the substrate, which limits its utility for many applications. Control over the position of MoS 2 flakes on oxidized silicon has been reported through the use of stamping [18] and masking [19] techniques, but neither of these allowed for the creation of large (tens of micrometres) monolayer domains at predetermined locations with micrometre-scale resolution. Substrate patterning has been used to control nucleation and growth of crystalline flakes of two-dimensional topological insulator materials on mica [20] , but it remains unclear whether this approach can be generalized to MoS 2 on oxidized silicon. Seeding techniques that allow growth at defined locations are well established for graphene [21] , [22] , and equivalent approaches for MoS 2 synthesis are highly desirable. Here we report the use of lithographically patterned islands of MoO 3 or ammonium heptamolybdate (AHM) as seed material for the growth of crystalline MoS 2 monolayers at predefined locations on oxidized silicon substrates. MoS 2 grown by this approach shows many favourable characteristics, for example, high crystallinity; excellent optical properties, including a direct bandgap, as indicated by photoluminescence (PL) and reflection measurements; and carrier mobility ca 10 cm 2 V −1 s −1 . Because the method enables control over the location of discrete MoS 2 flakes, integration into device structures is straightforward using optical lithography, with no need for an etching step. Although some applications may require further study to achieve control over the precise shape and size of the MoS 2 flakes, the methodology presented here opens a path towards scalable production of high-quality devices and circuits based on MoS 2 and other transition metal dichalcogenides. 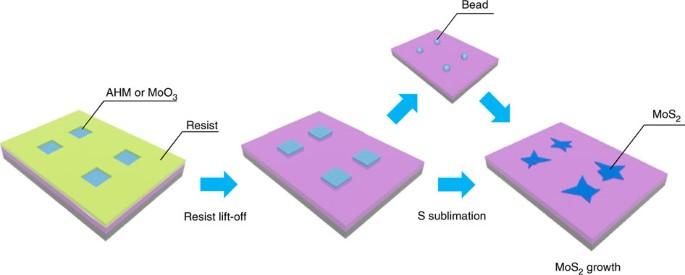Figure 1: Schematic of the growth process for molybdenum disulphide using patterned molybdenum sources. An array of square wells is patterned in a conventional lithographic resist. The wells are filled by spin coating with ammonium heptamolybdate ((NH4)6Mo7O24·4H2O, AHM) solution or thermal evaporation of molybdenum trioxide (MoO3). The resist is removed in a lift-off process. Water droplets are condensed onto the AMH or MoO3by reducing the sample temperature to below the dew point using a Peltier cooler. The AMH or MoO3is solubilized and forms spherical beads upon drying. MoS2flakes are then synthesized by sublimation of solid S in a nitrogen environment in a tube furnace. Growth process Figure 1 is a schematic of the MoS 2 growth process (see the Methods section and Supplementary Fig. 1 for details). The process begins with patterning of an array of square windows, typically 5–10 μm on a side, by e-beam or optical lithography. Next, molybdenum-containing seed material is deposited into the windows, either by thermal evaporation of MoO 3 or by spin-casting of a saturated solution of AHM in water. The AHM solution collects in the square wells but there is almost no deposition of AHM on the resist layer, which is not wet by the solution. Spin coating of AHM has advantages of speed, simplicity and requiring no equipment beyond a standard spin coater. The resist and unwanted molybdenum source material are removed in a standard lift-off step. Figure 1: Schematic of the growth process for molybdenum disulphide using patterned molybdenum sources. An array of square wells is patterned in a conventional lithographic resist. The wells are filled by spin coating with ammonium heptamolybdate ((NH 4 ) 6 Mo 7 O 24 ·4H 2 O, AHM) solution or thermal evaporation of molybdenum trioxide (MoO 3 ). The resist is removed in a lift-off process. Water droplets are condensed onto the AMH or MoO 3 by reducing the sample temperature to below the dew point using a Peltier cooler. The AMH or MoO 3 is solubilized and forms spherical beads upon drying. MoS 2 flakes are then synthesized by sublimation of solid S in a nitrogen environment in a tube furnace. Full size image At this point, the molybdenum-containing seed particle has a shape that depends upon the relative humidity and other details of the deposition process. To improve the uniformity of the seed shape and subsequent MoS 2 growth, an aggregation step is performed (see Supplementary Figs 2 and 3 ) where the sample temperature is reduced to below the dew point using a Peltier cooler. Owing to the hygroscopic nature of MoO 3 and AHM, water collects on the surface of the seed, which is transformed into a spherical-cap shape. This reduces the surface area of the seed particles and makes them more uniform, leading to more efficient and reproducible MoS 2 growth. This step ensures that the seed particle is sufficiently thick to not be consumed by evaporation during the heat-up phase of the growth process. This step is essential when AHM is used as the moblydenum source, as it is quite thin when initially deposited (~50 nm, see Supplementary Fig. 2 ). In contrast, the aggregation step improves the growth reproducibility but is not required when evaporation is used to deposit a MoO 3 seed of thickness approximately 150 nm or greater. The aggregation step is followed by an annealing step at 300 °C in a nitrogen atmosphere, which converts AHM to MoO 3 (refs 23 , 24 ). The next step in the process is chemical treatment of the SiO 2 surface, which has been shown to facilitate growth of MoS 2 . For example, it was reported that MoS 2 growth was promoted when the SiO 2 surface was coated with materials that contain carbon ring structures that persist at the MoS 2 growth temperature, for example, perylene-3,4,9,10-tetracarboxylicdianhydride, perylene-3,4,9,10-tetracarboxylic acid tetrapotassium salt [13] or reduced graphene oxide [13] , [16] . These materials promote monolayer growth by increasing the surface adhesive energy relative to the adatom cohesive energy [17] . We achieved excellent results by first preparing the surface with an oxygen plasma treatment and then spin-casting onto the substrate an aqueous solution of 0.1–1% sodium cholate, which contains multiple carbon ring structures. For MoS 2 growth, the sample was placed in the middle of the furnace, and 20–50 mg of solid sulphur was placed at the upstream end. The entire growth process, including temperature ramp, growth and cooling, was conducted under a nitrogen flow of 700 s.c.c.m. The use of patterned molybdenum source material resulted in the growth of an array of triangular/spike-shaped flakes of monolayer MoS 2 ( Figs 2a and 3a,b,d ). The flakes comprised multiple crystalline domains of MoS 2 , as analysed below (see Fig. 4 ). The majority of the flake region consisted of monolayer MoS 2 , with small regions of multilayer MoS 2 and/or residual seed material observed at the centre of the flake ( Fig. 3d ). It was found that the formation of multilayer regions could be suppressed by optimizing the dimensions of the growth seed (see Supplementary Fig. 4 ). The structure is consistent with a model where growth is initiated at multiple points on the MoO 3 seed to produce MoS 2 crystallites that eventually merge into a larger, faceted structure. For additional data in support of this picture, see Supplementary Fig. 5 . Although the sizes and locations of the flakes were primarily determined by the array of the growth seeds, it was consistently observed that flakes that grew at the edge of the array were markedly smaller than those that grew in the middle. This is presumed to reflect diffusion of source material as the furnace temperature was increased that led to shrinkage of seed particles on the edge of the array. Particles in the centre of the array are more replenished than those at the edges because of the larger number of neighbouring particles. Once sulphur sublimation and transport into the furnace occurs, the larger source particles at the centre of the array grow larger MoS 2 flakes than the smaller source particles at the edges. In some experiments, small, triangular, presumably single-crystal MoS 2 flakes were observed to grow in the regions between the MoO 3 seeds (data not shown). This occurred during growths that were at higher temperature compared with the samples shown in Figs 2a and 3a , and where sulphur was introduced at a later time. Presumably, these conditions allowed for evaporation of Mo from the growth seed, which then reacted with the injected sulphur to form MoS 2 crystallites in regions between the seeds. 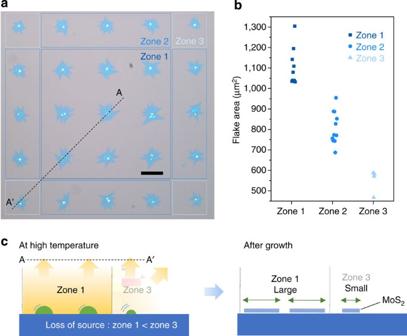Figure 2: Growth of molybdenum disulphide. (a) 5 × 5 array of flakes of monolayer MoS2grown by chemical vapour deposition. Scale bar is 50 μm. Different growth zones, with different average size of the flakes (seeb), are indicated by outlining: dark blue (zone 1), blue (zone 2) and light blue (zone 3). (b) Areas of individual flakes for zones 1, 2 and 3 ina. Large (500–1300 μm2) flakes of crystalline, monolayer MoS2(with small multilayer regions) were grown from the seed particles. The size of the flakes is largest in zone 1 and smallest in zone 3. (c) Schematic illustrating the proposed mechanism underlying the observation that the growth process results in larger MoS2flakes in the interior of the array and smaller flakes towards the edges. Figure 2: Growth of molybdenum disulphide. ( a ) 5 × 5 array of flakes of monolayer MoS 2 grown by chemical vapour deposition. Scale bar is 50 μm. Different growth zones, with different average size of the flakes (see b ), are indicated by outlining: dark blue (zone 1), blue (zone 2) and light blue (zone 3). ( b ) Areas of individual flakes for zones 1, 2 and 3 in a . Large (500–1300 μm 2 ) flakes of crystalline, monolayer MoS 2 (with small multilayer regions) were grown from the seed particles. The size of the flakes is largest in zone 1 and smallest in zone 3. ( c ) Schematic illustrating the proposed mechanism underlying the observation that the growth process results in larger MoS 2 flakes in the interior of the array and smaller flakes towards the edges. 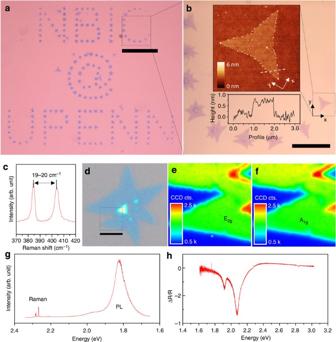Figure 3: AFM and optical analysis of MoS2flakes. (a) Optical micrograph of MoS2flakes grown at locations that form NBIC @ UPENN. Scale bar, 100 μm. (b) Selected area (dashed square ina) at higher magnification. Scale bar, 20 μm. Inset: AFM image of selected MoS2flake (dashed square). Scan image is 10 × 10 μm2. (c) Raman signal from the flake shows the E2gand A1gpeaks with a spacing (19 cm−1) characteristic of monolayer MoS2. (d) Optical image of MoS2flake from the array inFig. 2a. Scale bar, 10 μm. (e,f) 2D Raman maps taken from the flake shown ind(dashed line) for the E2gmode (e) and A1gmode (f). Scan images are 10 × 10 μm2. (g) Photoluminescence (PL) spectrum for the flake shows strong emission associated with the A and B excition at 1.83 eV and 1.97 eV, respectively. Strong PL is characteristic of monolayer MoS2and is absent in multilayer films. (h) Differential reflectance spectrum showing the A and B exciton features. Full size image Figure 3: AFM and optical analysis of MoS 2 flakes. ( a ) Optical micrograph of MoS 2 flakes grown at locations that form NBIC @ UPENN. Scale bar, 100 μm. ( b ) Selected area (dashed square in a ) at higher magnification. Scale bar, 20 μm. Inset: AFM image of selected MoS 2 flake (dashed square). Scan image is 10 × 10 μm 2 . ( c ) Raman signal from the flake shows the E 2g and A 1g peaks with a spacing (19 cm −1 ) characteristic of monolayer MoS 2 . ( d ) Optical image of MoS 2 flake from the array in Fig. 2a . Scale bar, 10 μm. ( e , f ) 2D Raman maps taken from the flake shown in d (dashed line) for the E 2g mode ( e ) and A 1g mode ( f ). Scan images are 10 × 10 μm 2 . ( g ) Photoluminescence (PL) spectrum for the flake shows strong emission associated with the A and B excition at 1.83 eV and 1.97 eV, respectively. Strong PL is characteristic of monolayer MoS 2 and is absent in multilayer films. ( h ) Differential reflectance spectrum showing the A and B exciton features. 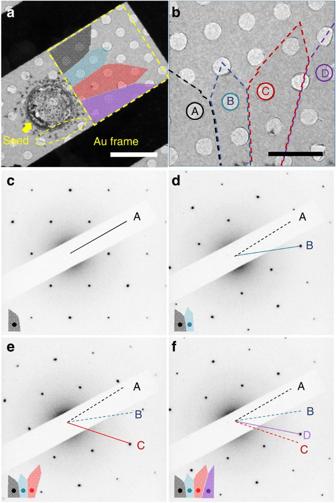Figure 4: Transmission electron micrographs and electron diffraction data. (a) Monolayer MoS2regions are coloured grey, light blue, red and purple (top-bottom) according to their crystallographic orientation. The black regions are parts of a gold frame used to prevent tearing during the transfer process (see main text andSupplementary Fig. 6). Triangular shaped multilayer MoS2flakes were formed in the seed region, indicated by the yellow arrow. (b) Bright-field (BF) image from the square region outlined by a dashed white line ina. Scale bars in figaandbare 5 μm and 3 μm, respectively. (c–f) Electron diffraction data from the regions labelled A–D inb. Full size image Figure 4: Transmission electron micrographs and electron diffraction data. ( a ) Monolayer MoS 2 regions are coloured grey, light blue, red and purple (top-bottom) according to their crystallographic orientation. The black regions are parts of a gold frame used to prevent tearing during the transfer process (see main text and Supplementary Fig. 6 ). Triangular shaped multilayer MoS 2 flakes were formed in the seed region, indicated by the yellow arrow. ( b ) Bright-field (BF) image from the square region outlined by a dashed white line in a . Scale bars in fig a and b are 5 μm and 3 μm, respectively. ( c – f ) Electron diffraction data from the regions labelled A–D in b . Full size image Structural and optical property measurements To demonstrate the versatility of the growth technique, we synthesized a set of monolayer MoS 2 flakes to spell out the acronym for the Nano-Bio Interface Center at the University of Pennsylvania, ‘NBIC@UPENN’ ( Fig. 3a ). The centre-to-centre spacing between adjacent seeds was ca 15 μm. Atomic force microscopy (AFM) was used to confirm that the height of a typical flake was 0.7 nm ( Fig. 3b , inset; additional line scan data are provided in Supplementary Fig. 6 . AFM images of other representative monolayer flakes of MoS 2 are provided in Supplementary Fig. 7 ), as expected for monolayer MoS 2 (refs 1 , 13 , 15 , 25 , 26 ). The Raman spectrum of the monolayer region of the flakes ( Fig. 3c ) showed the expected peak spacing of 19 cm −1 between the E 2g and A 1g modes. Raman mapping ( Fig. 3e,f ) was used to confirm that the Raman spectrum was uniform over the monolayer region as well as distinct from the spectra associated with multilayer regions and the substrate [25] , [26] , [27] (Maps of Raman peak positions are also shown in Supplementary Fig 8 . ). We performed PL and reflection measurements to confirm that the existence of a direct bandgap, which is known to be characteristic of monolayer MoS 2 (refs 28 , 29 , 30 , 31 ). Peak features associated with the A (1.83 eV in PL and 1.91 eV in reflection measurement) and B (1.97 eV in PL and 2.07 eV in reflection measurement) excitons were also observed ( Fig. 3f,g ), confirming that the MoS 2 grown by the seeded CVD process shows the same characteristics as monolayer material fabricated by mechanical exfoliation [32] . Sample crystallinity was further characterized with bright-field imaging and selected area electron diffraction (SAED) measurements conducted in the transmission electron microscope (TEM). A gold grid was first patterned onto a MoS 2 flake to prevent tearing of the flake when it was transferred onto a TEM grid covered by a carbon membrane with 1-μm diameter holes ( Fig. 4a and Supplementary Fig. 9 ). To minimize damage to the sample, imaging and SAED were conducted using an accelerating voltage of 80 kV. The TEM bright-field images are shown in Fig. 4a,b . Triangular shaped multilayer MoS 2 flakes were observed very close to the seed particle, possibly due to limited diffusion of the source during the growth time. Further from the seed, flower-petal-like monolayer MoS 2 regions were observed (dashed square in Fig. 4a,b ; see Supplementary Fig. 10 for the raw image used to create Fig. 4b and an atomic resolution image of a monolayer MoS 2 flake). The crystalline structure of the MoS 2 was investigated by SAED. Using the intensities of the first- and/or second-order diffraction spots [33] , [34] , the flower-petal-like structures were identified as monolayer MoS 2 (see Supplementary Fig. 11 ). Individual single-crystal MoS 2 domains, labelled A–D in Fig. 4b , were distinguished by the orientations of the diffraction spots in SAED ( Fig. 4c–f ). The data indicate that each domain is well crystallized and their orientations are uncorrelated. Fabrication and measurement of electronic devices An etch step is typically used to define individual devices from a continuous layer of material, which creates the risk of degrading a two-dimensional material as well as added processing cost. 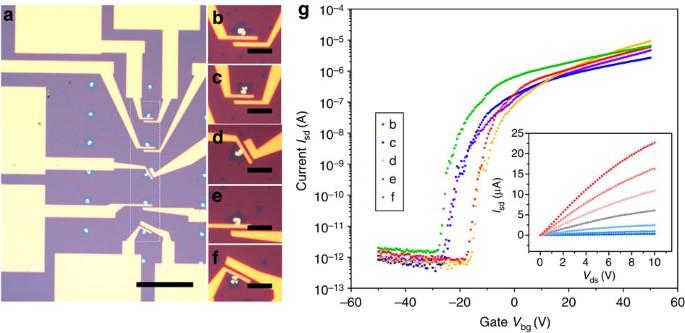Figure 5: Device fabrication andI–Vmeasurement. (a) Optical micrograph of devices that was fabricated from MoS2grown by the patterned seed technique. Scale bar, 100 μm. (b–f) Higher magnification images of the rectangular region indicated ina. Scale bar, 20 μm. (g)Ids–Vgcharacteristics for the devices inb–fwith 1 VVds. Inset:Ids–Vdscharacteristics at several back gate voltages. In contrast, the patterned growth approach to monolayer MoS 2 outlined here has the advantage of enabling direct fabrication of multiple devices ( Fig 5a–f ), without the need for etching. To demonstrate process compatibility with conventional manufacturing, an array of MoO 3 growth seeds was patterned by e-beam lithography, and MoS 2 monolayer flakes were synthesized as described above. As the MoS 2 flakes were grown at known, pre-patterned locations, it would be straightforward to align an electrode pattern to the MoS 2 flakes, with no need for a separate etch step. After fabrication of the electrodes, the sample was annealed at 150 °C at 10 −5 Torr for 1 h. Figure 5g shows the I ds – V g characteristics for a set of devices prepared using this approach, measured at a pressure of 40 mTorr. Device mobilities were between 8.2 and 11.4 cm 2 V −1 s −1 and the on/off ratios were in excess 10 6 comparable to earlier best reports for exfoliated MoS 2 monolayers [14] , [15] , [32] , [33] . Figure 5: Device fabrication and I – V measurement. ( a ) Optical micrograph of devices that was fabricated from MoS 2 grown by the patterned seed technique. Scale bar, 100 μm. ( b – f ) Higher magnification images of the rectangular region indicated in a . Scale bar, 20 μm. ( g ) I ds – V g characteristics for the devices in b – f with 1 V V ds . Inset: I ds – V ds characteristics at several back gate voltages. Full size image In summary, we have developed a novel patterned growth method for flakes of highly crystalline monolayer MoS 2 , where molybdenum-containing growth seeds (AHM or MoO 3 ) are defined using conventional lithographic methods. This technique should be generalizable to the growth of any layered transition metal dichalcogenide, and it creates a pathway to controllably tailor the size and position of the material. Control of growth parameters enables synthesis of high quality, crystalline, monolayer MoS 2 with electrical and optical properties comparable to exfoliated material. The process enables straightforward fabrication of integrated circuits without the need for a separate etch step. The work represents an important advance towards scalable production of high-quality layered transition metal dichalcogenide-based devices and circuits. An ongoing challenge to the field is patterned growth of monolayer, single-crystalline domain MoS 2 at predefined locations. Preparation of patterned molybdenum sources Electron beam or photolithography was used to prepare 5 × 5 arrays of 5-μm square windows. A 7 × 7 array of 3-μm square windows was used for the experiment that resulted in the growth of exclusively monolayer MoS 2 flakes (see Supplementary Fig. 4 ). Molybdenum-containing source material was then deposited by either spin coating (1,000 r.p.m. for 30 s, followed by 3,000 r.p.m. for 10 s) with a saturated solution of AHM (product number A674, Fisher Scientific) in deionized water or thermal evaporation of 150-nm-thick molybdenum trioxide (MoO 3 , product number 203815, Sigma-Aldrich). The resist was removed using acetone followed by isopropyl alcohol, and the sample was then blown dry with compressed nitrogen gas. An aggregation step was then performed to obtain regular beads of the source material. Although monitoring the sample under an optical microscope, the substrate was cooled until the hygroscopic AHM or MoO 3 absorbed water, forming droplets at the seed locations. As the temperature was increased back to room temperature, the water evaporated, leaving behind rounded, uniform, beads of AHM or MoO 3 as shown in Supplementary Fig. 2 . Samples were then annealed at 300 °C for 20 min in a flow of 500 s.c.c.m. of nitrogen gas (99.999% purity). To promote MoS 2 growth, the sample was treated with oxygen plasma (65 W, 300 mTorr, 2 min) and then spin-coated (3,000 r.p.m., 1 min) with a surfactant solution (0.1–1% solution of sodium cholate in deionized water). Growth process Samples with patterned growth seeds were placed into a 1-inch CVD furnace with a 25-mg solid sulphur source (part number 213292, Sigma-Aldrich) at the upstream end. The furnace temperature was increased to 750 °C at a ramp rate of 70 °C min −1 under a nitrogen (99.999%) flow of 700 s.c.c.m. The temperature was held constant for 20 min during the MoS 2 growth phase, and the system was then rapidly cooled to room temperature. It was noted that the sulphur source started to melt when the temperature in the middle of the furnace was ca 650 °C. Device fabrication and current–voltage measurements After growth of monolayer MoS 2 flakes from patterned growth seeds, electron beam lithography was used to define an electrode pattern that was aligned to the growth sites. The electrode metallization consisted of 1 nm Cr and 30 nm Au deposited by e-beam evaporation. After metallization, devices were annealed for 60 min at 150 °C at a pressure of 10 −5 Torr. Current–voltage measurements were conducted at room temperature under a vacuum of 40 mTorr. How to cite this article: Han, G. H. et al . Seeded growth of highly crystalline molybdenum disulphide monolayers at controlled locations. Nat. Commun. 6:6128 doi: 10.1038/ncomms7128 (2015).